Weak functional group interactions revealed through metal-free active template rotaxane synthesis Modest functional group interactions can play important roles in molecular recognition, catalysis and self-assembly. However, weakly associated binding motifs are often difficult to characterize. Here, we report on the metal-free active template synthesis of [2]rotaxanes in one step, up to 95% yield and >100:1 rotaxane:axle selectivity, from primary amines, crown ethers and a range of C=O, C=S, S(=O) 2 and P=O electrophiles. In addition to being a simple and effective route to a broad range of rotaxanes, the strategy enables 1:1 interactions of crown ethers with various functional groups to be characterized in solution and the solid state, several of which are too weak — or are disfavored compared to other binding modes — to be observed in typical host–guest complexes. The approach may be broadly applicable to the kinetic stabilization and characterization of other weak functional group interactions. The bulky axle end-groups of rotaxanes mechanically lock rings onto threads, preventing the dissociation of the components even if the interactions between them are not strong and attractive [1] , [2] , [3] . In principle the enforced high local concentration of convergent functional groups brought about by such mechanical bonding can stabilize weak non-covalent interactions [4] . In practice such outcomes are rarely observed [4] , [5] , [6] , [7] , [8] because most rotaxane syntheses rely upon strong attractive interactions between the building blocks [2] , [3] , [9] , [10] , [11] , [12] , [13] to promote the rotaxane assembly process. Strong binding modes generally ‘live on’ in the interlocked product, an outcome useful for the design of artificial molecular machinery [2] , [3] , [14] , [15] , [16] , whether intended to operate in solution [17] or when organized on surfaces [18] , [19] or within metal-organic frameworks [20] , [21] , but one that tends to override alternative weaker binding modes that could occur between the components. It is sometimes possible to remove strong template interactions by post-assembly modification, for example by deprotonation of an ammonium unit [22] , [23] , but this is often not straightforward and can require forcing conditions [23] . Active template synthesis [24] , [25] , [26] , [27] , [28] , [29] , [30] , [31] , [32] , [33] , [34] , [35] , in which a macrocycle accelerates a strand-forming reaction through the ring cavity, does not require strong pre-association of the starting materials. Although most active template syntheses have been developed from transition metal catalyzed reactions [24] , [25] , [26] , [27] , [28] , [29] , [30] , [31] , [32] , [33] , [34] , [35] , a metal-free active template system was recently discovered [36] , [37] in which the addition of primary amines to electrophiles can be significantly accelerated through crown ethers [37] and related macrocycles [36] by stabilization of the reaction transition state [38] , [39] , [40] , [41] , [42] , [43] . The reaction of a primary amine and an electrophile in the presence of a crown ether was found [37] to form [2]rotaxanes by metal-free active template N -alkylation, aza-Michael addition or N -acylation. In these reactions the crown ether stabilizes developing partial charges in the transition state causing initial rate accelerations of up to 26× through the macrocycle compared with the reaction exo- to the cavity that forms the non-interlocked axle. The N -acylation reaction is particularly effective: simply mixing together 1.0 equivalents of each of 24-crown-8 1 , amine 2 , and activated ester 3 in toluene at room temperature spontaneously assembles amide-axle [2]rotaxane 4 in 56% yield, without the need for any other reagents or excess building blocks (Fig. 1 ). This potentially offers access to kinetically locked systems with unusual combinations of functional groups on the different components forced into close proximity and a 1:1 stoichiometry. The interaction of the groups on different components might further be enhanced by the tendency of interlocked architectures to have poorly solvated inner surfaces. Fig. 1: N -Acylation active template rotaxane synthesis. The yield of rotaxane is increased by addition of Et 3 N to neutralize the acidic phenolic byproduct of the reaction or the use of less nucleophilic primary amine 5 . Full size image To explore the scope of this unexpected method of rotaxane synthesis, here we carry out a study of the reaction with a series of related electrophiles. After developing an optimized set of reaction conditions, rotaxanes were accessed by crown ether-stabilized formation of (thio)urea, carbamate, sulfonamide, and phosphoramidate/phosphinamide-containing axles. The stabilization of S N Ar reactions between primary amines and electron-deficient aryl halides led to rotaxanes with aniline threads. Single-crystal X-ray diffraction of the rotaxanes enabled weak interactions between the crown ether and the newly formed functional groups in the axles to be studied. Optimization of metal-free active template rotaxane synthesis by N -acylation Complete consumption of crown ether 1 does not occur with the experimental protocol originally used for the active template N -acylation rotaxane-forming reaction (Fig. 1 ), even with a fivefold excess of amine 2 . Proton nuclear magnetic resonance ( 1 H NMR) showed that rotaxane 4 is initially formed rapidly, but over time its rate of formation slows relative to the background reaction of amine and ester, resulting in increasing amounts of non-interlocked axle. The color change that occurs during the early stages of that reaction suggested that liberation of the yellow 4-nitrophenolate anion [44] might be inhibiting the formation of rotaxane 4 . We reasoned that 4-nitrophenol, formally the other product of the N -acylation reaction, would be deprotonated by 2 and the resulting primary ammonium cation ( 2 H + ) would bind strongly to the crown ether preventing it from participating in the active template reaction. 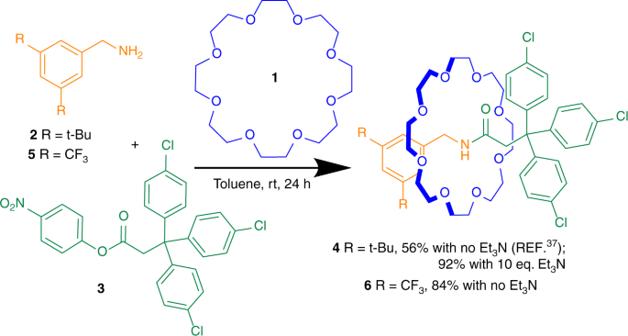Fig. 1:N-Acylation active template rotaxane synthesis. The yield of rotaxane is increased by addition of Et3N to neutralize the acidic phenolic byproduct of the reaction or the use of less nucleophilic primary amine5. Accordingly, we investigated whether the yield of 4 could be improved by the addition of tertiary amines, which when protonated bind more weakly to crown ethers than primary ammonium salts [45] (Supplementary Table 1 ). Pleasingly, addition of 10 equivalents (equiv.) of triethylamine (Et 3 N) led to the formation of rotaxane 4 in 68% yield after 1 h and 92% yield after 24 h. Under these conditions the ratio of rotaxane 4 to non-interlocked axle improved from 8:1 to 17:1 after 24 h, indicating that Et 3 N does not promote aminolysis of the building blocks in the absence of the crown ether. In contrast, the use of a stronger base, 1,8-diazabicyclo[5.4.0]undec-7-ene (DBU), significantly reduced the formation of 4 (10% yield after 1 h) while increasing the amount of non-interlocked axle formed, suggesting that DBU accelerates the reaction of 2 and 3 at the expense of the active template reaction [46] , [47] , [48] . 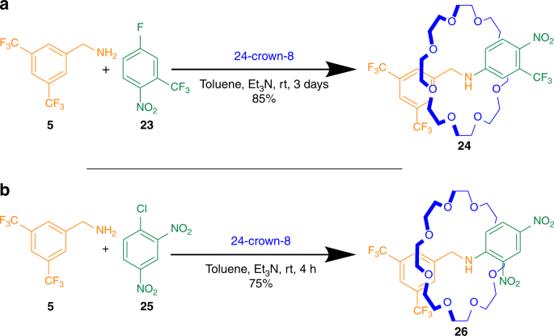Fig. 2:N-Arylation active template rotaxane synthesis. Rotaxanes containing aniline axles could be obtained by the SNAr reaction between primary amine5andaaryl fluoride23orbaryl chloride25. We next investigated the efficacy of rotaxane formation with less nucleophilic benzylic amines (Supplementary Table 2 ). Commercially available amine 5 , bearing two CF 3 substituents, proved the most effective amine tested, with [2]rotaxane 6 formed in 84% yield after 24 h without the need for Et 3 N (Fig. 1 ), with a rotaxane:non-interlocked axle ratio >100:1 (determined by 1 H NMR). This remarkable selectivity for acylation through the cavity appears to be a consequence of the background acylation reaction (to form the non-interlocked axle) having an activation energy in the ‘sweet spot’ for active template synthesis: too high for acylation to occur quickly with the less nucleophilic amine ( 5 ) but low enough that a few kcal mol −1 stabilization of the transition state by the crown ether brings about a very significant rate enhancement. 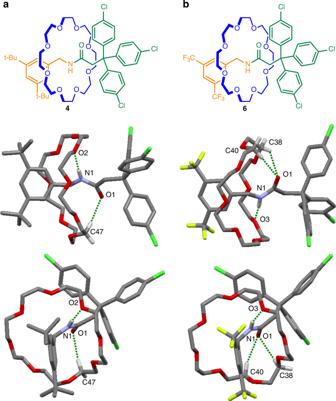Fig. 3: X-ray crystal structures of crown ether–amide-axle rotaxanes. aRotaxane4. Hydrogen bond lengths [Å]: O1—H47C, 2.47; O2—H1N, 2.12. Hydrogen bond angles (deg): O1—H47C, 166.3; O2—H1N, 173.1.bRotaxane6. Hydrogen bond lengths [Å]: O1—H38C, 2.48; O1—H40C, 2.55; O3—H1N, 2.20. Hydrogen bond angles (deg): O1—H38C, 129.5; O1—H40C, 161.0; O3—H1N, 163.0. NH···O and CH···O hydrogen bonds shown in dark green. Solvate molecules and other hydrogen atoms omitted for clarity. It also proved possible to use more reactive electrophiles with amine 5 (Supplementary Table 3 ). Rotaxane 6 was obtained in 54% yield from the corresponding acid chloride and in 40% yield when using the 1-hydroxybenzotriazole ester as the electrophile. C=O/C=S/SO 2 /P=O electrophile scope With improved conditions for active template ester aminolysis in hand we investigated whether the type of rotaxanes accessible could be expanded upon using electrophiles based on different, but structurally related, chemical functionality ( 7 – 14 , Table 1 ). 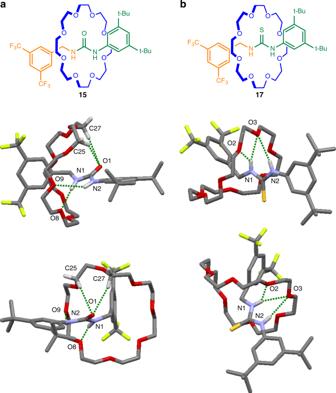Fig. 4: X-ray crystal structures of crown ether urea and thiourea axle rotaxanes. aRotaxane15. Hydrogen bond lengths [Å]: O1—H25C, 2.66; O1-H27C, 2.71; O8—H1N, 2.12; O9—H2N, 2.65. Hydrogen bond angles (deg): O1—H25C, 145.4; O1-H27C, 165.0; O8—H1N, 169.7; O9—H2N, 143.2.bRotaxane17. Hydrogen bond lengths [Å]: O2—H1N, 2.41; O3—H1N, 2.32; O3—H2N, 2.74. Hydrogen bond angles (deg): O2—H1N, 126.9; O3—H1N, 158.3; O3—H2N, 148.5. NH···O and CH···O hydrogen bonds shown in dark green. Solvate molecules and other hydrogen atoms omitted for clarity. The aminolysis of carbamates [49] follows a similar mechanistic pathway to ester aminolysis: nucleophilic attack at the carbonyl forms a tetrahedral intermediate followed by loss of the leaving group to form urea [50] , [51] , [52] . Accordingly we tested whether carbamate 7 was a suitable electrophile for the metal-free active template reaction. Reaction of 7 , amine 5 and 24-crown-8 1 in a 1:1:1 ratio, under the standard reaction conditions (without Et 3 N), afforded urea [2]rotaxane 15 in 73% yield (Table 1 , entry 1). Urea rotaxane formation was also possible without generating a leaving group byproduct through the use of isocyanate 8 , which gave rotaxane 16 in 55% yield (Table 1 , entry 2). The reaction between 5 and 8 proceeded extremely quickly; full conversion of 5 was achieved within 1 min. The corresponding thiourea rotaxane 17 was prepared in an analogous manner from isothiocyanate 9 in 54% yield (Table 1 , entry 3). Table 1 Synthesis of [2]rotaxanes from 24-crown-8, amine 5 and C=O/C=S/SO 2 /P=O electrophiles 7 – 14 a Full size table Carbamate rotaxanes were accessible using common commercially available electrophiles. Activated carbonate 10 , used to form carbamates that can be readily decomposed with fluoride [53] , gave 18 in 83% yield (Table 1 , entry 4), while chloroformate 11 (Fmoc-Cl) generated 19 in 70% yield with Et 3 N added to neutralize the HCl product (Table 1 , entry 5) [54] . The ability to release the macrocycle from these types of rotaxanes in response to a specific chemical stimulus (stoichiometric fluoride for 18 ; catalytic base for 19 ) may prove useful for future applications. Electrophiles containing a heteroatom at the site of nucleophilic attack also proved effective for rotaxane formation. Sulfonyl chloride 12 , a bulky analog of tosyl chloride, reacted with 5 and 1 to give sulfonamide rotaxane 20 in 95% yield (Table 1 , entry 6). Diphenyl phosphoryl chloride 13 produced phosphoramidate rotaxane 21 in 90% yield (Table 1 , entry 7), while the more reactive diphenyl phosphinic chloride 14 resulted in the formation of phosphinamide rotaxane 22 in a more modest 29% yield (Table 1 , entry 8). As the sulfur and phosphorus electrophiles feature chloride leaving groups, in each case Et 3 N was added to neutralize the HCl formally released by the active template reaction. Metal-free active template synthesis by N -arylation To further expand on the general applicability of active template rotaxane synthesis with crown ethers, we explored other potential reaction modes. Prompted by a recent report [55] of crown ether catalysis of S N Ar reactions between aryl halides and primary amines, we investigated rotaxane formation by N -arylation. This proved effective using different electrophiles: combining amine 5 and 24-crown-8 1 with aryl fluoride 23 in the presence of Et 3 N produced aniline rotaxane 24 in 85% yield (Fig. 2a ), while combining 5 and 1 with aryl chloride 25 formed aniline rotaxane 26 in 75% yield (Fig. 2b ). Both rotaxanes were isolated as neutral amines rather than as the corresponding ammonium salts. As the p K a values of protonated anilines are readily modulated by changing the aromatic substitution [56] , rotaxanes such as 24 and 26 have the potential to be used as tunable pH-sensitive molecular switches of basicity lower than that of commonly used dibenzylammonium-crown ether systems [3] . 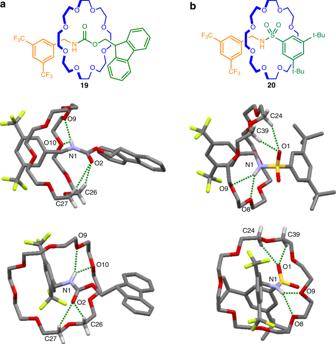Fig. 5: X-ray crystal structures of crown ether carbamate and sulfonamide axle rotaxanes. aRotaxane19. Hydrogen bond lengths [Å]: O2—H26C, 2.53; O2—H27C, 2.88; O9—H1N, 2.27; O10—H1N, 2.65. Hydrogen bond angles (deg): O2—H26C, 155.4; O2—H27C, 142.7; O9—H1N, 154.4; O10—H1N, 135.0.bRotaxane20. Hydrogen bond lengths [Å]: O1—H24C, 2.50; O1—H39C, 2.64; O8—H1N, 2.31; O9—H1N, 2.61. Hydrogen bond angles (deg): O1—H24C, 149.3; O1—H39C, 144.8; O8—H1N, 145.6; O9—H1N, 144.9. NH···O and CH···O hydrogen bonds shown in dark green. Solvate molecules and other hydrogen atoms omitted for clarity. 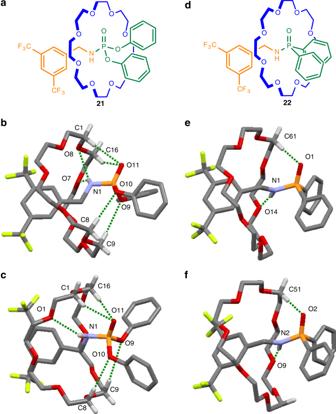Fig. 6: X-ray crystal structures of crown ether phosphoramidate and phosphinate axle rotaxanes. aRotaxane21. The hydrogen atom bonded to N1in21is disordered over two positions, each structure is shown in (b) and (c).bHydrogen bond lengths [Å]: O9—H9C, 3.14; O10—H8C, 2.75; O11—H1C, 2.52; O11—H16C, 2.60; O7—H1N, 2.71; O8—H1N, 2.62. Hydrogen bond angles (deg): O9—H9C, 165.3; O10—H8C, 168.2; O11—H1C, 152.5; O11—H16C, 146.1; O7—H1N, 157.7; O8—H1N, 134.0.cHydrogen bond lengths [Å]: O1—H1N, 2.65; O9—H9C, 3.14; O10—H8C, 2.75; O11—H1C, 2.52; O11—H16C, 2.60. Hydrogen bond angles (deg): O1—H1N, 144.2; O9—H9C, 165.3; O10—H8C, 168.2; O11—H1C, 152.5; O11—H16C, 146.1.dRotaxane22. Two co-conformations of22co-crystallize, each is shown in (e) and (f).eHydrogen bond lengths [Å]: O1—H61C, 2.39; O14—H1N, 2.36. Hydrogen bond angles (deg): O1—H61C, 171.5; O14—H1N, 174.3.fHydrogen bond lengths [Å]: O2—H51C, 2.37; O9—H2N, 2.41. Hydrogen bond angles (deg): O2—H51C, 172.5; O9—H2N, 175.1. NH···O and CH···O hydrogen bonds shown in dark green. Solvate molecules and other hydrogen atoms omitted for clarity. Fig. 2: N -Arylation active template rotaxane synthesis. Rotaxanes containing aniline axles could be obtained by the S N Ar reaction between primary amine 5 and a aryl fluoride 23 or b aryl chloride 25 . Full size image Crown ether-functional group interactions Complexes between crown ethers and neutral molecules were first reported by Pedersen nearly 50 years ago [57] , with the majority of examples described to date involving relatively small macrocycles such as 18-crown-6 (refs. [58] , [59] , [60] , [61] ). Neutral molecules cannot be fully encapsulated within such small cavities and so the complexes tend to be of a ‘perch’ type. With such binding modes the crown ethers often bind to more than one guest to maximize favorable host–guest interactions and to balance the dipole moments of polar guests. In the solid state discrete 1:1 crown ether–neutral molecule complexes are rare and a range of different binding modes and ratios can sometimes be observed with only minor variations in structure arising from different crystallization conditions [59] , [60] , [61] . In contrast to such host–guest complexes, the interlocked components of rotaxanes have a strictly defined stoichiometry (usually 1:1), are held in close proximity, and possess limited co-conformational [62] degrees of freedom [63] , [64] , [65] , [66] , [67] , [68] , [69] , [70] , [71] . In the absence of strong binding between the components weak interactions that are seldom observable in supramolecular complexes can form and significantly influence co-conformation [4] , [5] . Rotaxanes 4 , 6 , 15 , 17 , and 19 – 22 provide architectures in which functional groups in the axle are mechanically locked through the crown ether ring in a 1:1 stoichiometry, enabling normally weak interactions to be characterized experimentally. Slow evaporation of CH 2 Cl 2 /hexane solutions of 4 , 17 , 21 , and 22 , and of diethyl ether/hexane solutions of 6 , 15 , 19 , and 20 afforded single crystals suitable for X-ray diffraction of rotaxanes containing each of the axle functionalities formed through metal-free active template synthesis. X-ray crystal structures of [2]rotaxanes 4 and 6 In structures in the Cambridge Crystallographic Data Centre (CCDC) database, crown ether–amide host–guest binding typically occurs with a 1:2 stoichiometry, with the crown ether oxygen atoms accepting hydrogen bonds from the amide guest [57] , [58] , [59] , [60] . In the amide-axle rotaxanes 4 and 6 (Fig. 3 ) a 1:1 crown ether:amide interaction stoichiometry occurs and in each structure a crown ether oxygen hydrogen bonds to the amide hydrogen atom while CH …. O hydrogen bonds stabilize the electron density on the amide oxygen atom [72] , [73] . The O …. H–N hydrogen bond in 4 is shorter than in 6 (O …. H distances: 2.12 Å ( 4 ); 2.20 Å ( 6 )), despite the electron-withdrawing CF 3 groups in 6 . In 4 the oxygen interacts with a single C–H group (O …. H distance: 2.47 Å), while in 6 three-centered bifurcated hydrogen bonding occurs between the carbonyl oxygen and two C–H groups (O …. H distances: 2.48 and 2.55 Å) [74] . Such CH …. O hydrogen bonding is reminiscent of interactions within peptide chains that stabilize protein secondary structure [75] . Fig. 3: X-ray crystal structures of crown ether–amide-axle rotaxanes. a Rotaxane 4 . Hydrogen bond lengths [Å]: O1—H47C, 2.47; O2—H1N, 2.12. Hydrogen bond angles (deg): O1—H47C, 166.3; O2—H1N, 173.1. b Rotaxane 6 . Hydrogen bond lengths [Å]: O1—H38C, 2.48; O1—H40C, 2.55; O3—H1N, 2.20. Hydrogen bond angles (deg): O1—H38C, 129.5; O1—H40C, 161.0; O3—H1N, 163.0. NH···O and CH···O hydrogen bonds shown in dark green. Solvate molecules and other hydrogen atoms omitted for clarity. Full size image X-ray crystal structures of [2]rotaxanes 15, 17, and 19 Crown ethers and (thio)ureas tend to form complex extended networks in the solid state, with the ratio of host-to-guest varying significantly and unpredictably [57] . In contrast rotaxanes 15 , 17 , and 19 form discrete structures with 1:1 crown ether:urea/thiourea association. Rotaxanes 15 and 17 (Fig. 4 ) each contain two different types of N–H groups: one nitrogen atom conjugated to an aromatic ring, the other benzylic. In both solid state structures the crown ether forms shorter hydrogen bonds with the benzylic N–H group. In 15 the interaction occurs with a single crown ether oxygen (O …. H distance: 2.12 Å), while a bifurcated hydrogen bond occurs with two oxygen atoms in 17 (O …. H distances: 2.32 and 2.41 Å). An additional long hydrogen bond from an ether oxygen to the other NH group is present in both rotaxanes (O …. H distances: 2.65 and 2.74 Å for 15 and 17 , respectively). A bifurcated hydrogen bond between two crown ether oxygens and the N–H moiety of the carbamate group (O …. H distances: 2.27 and 2.65 Å) occurs in 19 . The slightly longer O …. HN bond lengths in 19 (Fig. 5 ) versus 15 are consistent with the weaker hydrogen bond-donating ability of a carbamate group compared with urea [76] , [77] . Similar to an amide group, the carbonyl oxygens act as hydrogen bond acceptors from C–H groups of the crown ether in 15 and 19 , with bifurcated hydrogen bonds formed in both cases (O …. H distances: 2.66 and 2.71 Å for 15 ; 2.53 and 2.88 Å for 19 ). The sulfur atom in 17 does not engage in a similar interaction reflecting the more modest hydrogen bond basicity of thioureas [78] . Fig. 4: X-ray crystal structures of crown ether urea and thiourea axle rotaxanes. a Rotaxane 15 . Hydrogen bond lengths [Å]: O1—H25C, 2.66; O1-H27C, 2.71; O8—H1N, 2.12; O9—H2N, 2.65. Hydrogen bond angles (deg): O1—H25C, 145.4; O1-H27C, 165.0; O8—H1N, 169.7; O9—H2N, 143.2. b Rotaxane 17 . Hydrogen bond lengths [Å]: O2—H1N, 2.41; O3—H1N, 2.32; O3—H2N, 2.74. Hydrogen bond angles (deg): O2—H1N, 126.9; O3—H1N, 158.3; O3—H2N, 148.5. NH···O and CH···O hydrogen bonds shown in dark green. Solvate molecules and other hydrogen atoms omitted for clarity. Full size image Fig. 5: X-ray crystal structures of crown ether carbamate and sulfonamide axle rotaxanes. a Rotaxane 19 . Hydrogen bond lengths [Å]: O2—H26C, 2.53; O2—H27C, 2.88; O9—H1N, 2.27; O10—H1N, 2.65. Hydrogen bond angles (deg): O2—H26C, 155.4; O2—H27C, 142.7; O9—H1N, 154.4; O10—H1N, 135.0. b Rotaxane 20 . Hydrogen bond lengths [Å]: O1—H24C, 2.50; O1—H39C, 2.64; O8—H1N, 2.31; O9—H1N, 2.61. Hydrogen bond angles (deg): O1—H24C, 149.3; O1—H39C, 144.8; O8—H1N, 145.6; O9—H1N, 144.9. NH···O and CH···O hydrogen bonds shown in dark green. Solvate molecules and other hydrogen atoms omitted for clarity. Full size image X-ray crystal structures of [2]rotaxanes 20–22 In the solid state rotaxanes 20 , 21 , and 22 all have rather similar intercomponent interactions to each other. In supramolecular complexes, sulfonamides usually bind to crown ethers through hydrogen bonds donated by the N–H group [79] . In the X-ray crystal structure of 20 the N–H forms a bifurcated hydrogen bond with two crown ether oxygens (O …. H distances: 2.31 and 2.61 Å; Fig. 5 ). Another bifurcated hydrogen bond is formed between two C–H groups of the crown ether and a single sulfonamide oxygen (O …. H distances: 2.50 and 2.64 Å). The crown ether does not adopt a conformation that enables simultaneous interactions with both sulfonamide oxygens [80] . Phosphorous analogs of amides often form intermolecular P–O …. H–N hydrogen bonds in the solid state, driven by the particularly strong hydrogen bond accepting ability of P=O [76] , [81] . However, as with the other rotaxanes described in this series, intermolecular interactions between axles is inhibited in 21 and 22 by encapsulation of the phosphoramidate and phosphinate units by the crown ether [82] , [83] . The N–H hydrogen atom in 21 (Fig. 6 ) is disordered over two positions, while the sp 2 -hybridized oxygen forms a bifurcated hydrogen bond with two crown ether C–H groups (O …. H distances: 2.52 and 2.60 Å). The sp 3 -hybridized oxygen atoms bound to phosphorous each form relatively long hydrogen bonds with a single C–H group of the crown ether (O …. H distances: 2.75 and 3.14 Å). Two conformations of 22 co-crystallize, both with a single ether oxygen forming a hydrogen bond with the N–H group (average O …. H distance 2.39 Å) and a single hydrogen bond between the phosphinyl oxygen atom and a C–H group of the crown ether (average O …. H distance 2.38 Å). Fig. 6: X-ray crystal structures of crown ether phosphoramidate and phosphinate axle rotaxanes. a Rotaxane 21 . The hydrogen atom bonded to N 1 in 21 is disordered over two positions, each structure is shown in ( b ) and ( c ). b Hydrogen bond lengths [Å]: O9—H9C, 3.14; O10—H8C, 2.75; O11—H1C, 2.52; O11—H16C, 2.60; O7—H1N, 2.71; O8—H1N, 2.62. Hydrogen bond angles (deg): O9—H9C, 165.3; O10—H8C, 168.2; O11—H1C, 152.5; O11—H16C, 146.1; O7—H1N, 157.7; O8—H1N, 134.0. c Hydrogen bond lengths [Å]: O1—H1N, 2.65; O9—H9C, 3.14; O10—H8C, 2.75; O11—H1C, 2.52; O11—H16C, 2.60. Hydrogen bond angles (deg): O1—H1N, 144.2; O9—H9C, 165.3; O10—H8C, 168.2; O11—H1C, 152.5; O11—H16C, 146.1. d Rotaxane 22 . Two co-conformations of 22 co-crystallize, each is shown in ( e ) and ( f ). e Hydrogen bond lengths [Å]: O1—H61C, 2.39; O14—H1N, 2.36. Hydrogen bond angles (deg): O1—H61C, 171.5; O14—H1N, 174.3. f Hydrogen bond lengths [Å]: O2—H51C, 2.37; O9—H2N, 2.41. Hydrogen bond angles (deg): O2—H51C, 172.5; O9—H2N, 175.1. NH···O and CH···O hydrogen bonds shown in dark green. Solvate molecules and other hydrogen atoms omitted for clarity. Full size image Metal-free active template synthesis is a simple and versatile method through which to access crown ether rotaxanes with a discrete but diverse set of functionalities in the axle. The rotaxane assembly procedure is exceptionally simple, requiring only mixing of a crown ether, amine, and electrophile in toluene. All of the building blocks used in this paper are either currently commercially available or, in the case of amine 2 , ester 3 , carbamate 7 , isothiocyanate 9 , and sulfonyl chloride 12 , accessible in a single synthetic step. The rotaxane-forming reactions can be performed using a 1:1:1 stoichiometry of the three building blocks, in some cases generating rotaxanes in yields as high as 95% with >100:1 rotaxane:axle selectivity. In addition to being a simple and effective route to a wide range of rotaxanes the strategy enables 1:1 interactions of crown ethers with various functional group types to be characterized, several of which are too weak—or are disfavored compared with other binding modes—to be observed in conventional host–guest complexes. As of 23 September 2019 the CCDC contained >2000 X-ray crystal structures featuring crown ethers. The structures reported in this paper include the first few examples of crown ether–alkylsulfonamide, crown ether–phosphoramidate, crown ether–phosphonate, and crown ether–carbamate interactions, and only the second examples of crown ether–primary amide, crown ether-substituted urea, and crown ether-substituted thiourea interactions. Active template synthesis, essentially the use of catalysis to form and kinetically trap an unstable assembly, should prove to be a generally applicable tool for revealing weak functional group interactions. The difficulties in characterizing weak interactions was recently highlighted by Colizzi et al. [84] : “…intramolecular hydrogen bonds are widespread in biological molecules and are crucial in the design of new drugs and materials, including supramolecular machines… Unfortunately, the characterization of intramolecular H-bonds (and their utilization) is still limited, most likely as a consequence of the complexities that hamper the interpretation of experimental data obtained for large and flexible entities.” The ability to kinetically stabilize modest strength hydrogen bonding modes is another noteworthy consequence of the mechanical bond [3] . Synthesis of rotaxanes The synthesis and characterization of the rotaxanes and building blocks are provided in the Supplementary Methods. Representative synthesis of rotaxane 15 : To a stirring solution of 1 (49 mg, 0.14 mmol, 1.0 equiv.) and 5 (34 mg, 0.14 mmol, 1.0 equiv.) in toluene (1.0 mL) was added 7 (52 mg, 0.14 mmol, 1.0 equiv.). The mixture was stirred for 1 h and then concentrated under reduced pressure. Flash chromatography of the residue (SiO 2 , EtOAc/petroleum ether 1:5 then CH 2 Cl 2 /MeOH 50:1) afforded rotaxane 15 as a colorless solid (85 mg, 0.10 mmol, 73%).